Peptidomimetic targeting of critical androgen receptor–coregulator interactions in prostate cancer The growth of advanced prostate cancer depends on androgen receptor signalling, however treatment options are limited. Here we report the disruption of specific protein–protein interactions involving LXXLL motifs in androgen receptor–coregulator proteins such as PELP1 using a novel, small molecule peptidomimetic ( D2 ). D2 is stable, non-toxic and efficiently taken up by prostate cancer cells. Importantly, D2 blocks androgen-induced nuclear uptake and genomic activity of the androgen receptor. Furthermore, D2 abrogates androgen-induced proliferation of prostate cancer cells in vitro with an IC 50 of 40 nM, and inhibits tumour growth in a mouse xenograft model. D2 also disrupts androgen receptor–coregulator interactions in ex vivo cultures of primary human prostate tumours. These findings provide evidence that targeting androgen receptor–coregulator interactions using peptidomimetics may be a viable therapeutic approach for patients with advanced prostate cancer. The androgen receptor (AR) is a ligand-dependent transcription factor, which has a critical role in prostate cancer development and progression and is functionally active even in the late, terminal stages of the disease resistant to endocrine therapies, known as castration-resistant prostate cancer (CRPC) [1] , [2] . Chen et al . [3] , using transcript profiling of human prostate cancer xenografts, elegantly demonstrated that an increase in AR expression was consistently associated with the development of CRPC and that the increased level of AR was both necessary and sufficient to convert prostate cancer growth from hormone-sensitive to hormone-refractory. Importantly, functional AR signalling appears to be inappropriately restored in the castrate or androgen-deplete environment, including AR amplification and/or overexpression, gain-of-function AR mutations that facilitate ligand promiscuity or spliced variants that are constitutively active, intracrine androgen production, overexpression of AR coactivators, and indirect AR activation by growth factors, cytokines or aberrant AR phosphorylation [2] , [4] , [5] , [6] , [7] . These AR-dependent mechanisms highlight that a common feature of CRPC is an addiction to AR signalling [5] . Therefore, there remains a critical and unmet need for novel therapeutic agents that can directly target and inhibit the AR in advanced prostate cancer by means other than inhibiting androgen-induced activation. The AR predominantly resides in the cytoplasm until it is activated by its cognate ligands, testosterone or the more potent metabolite, 5α-dihydrotestosterone (DHT) [6] . Upon ligand binding, AR translocates to the nucleus and binds to androgen-responsive elements (ARE) in the regulatory regions of target genes, thereby modulating transcription. Through this genomic pathway, AR regulates the expression of more than a thousand genes, including the AR itself and well-characterized target genes such as prostate-specific antigen (PSA), to control the development and maintenance of the male phenotype [8] , [9] . Vital for AR-mediated transcription is the recruitment of AR coregulators and the transcriptional machinery [10] , [11] , [12] . Proline-, glutamic acid- and leucine-rich protein 1 (PELP1) is one such coregulator that serves as a scaffold between nuclear receptors such as AR and various signalling factors, including transcriptional, chromatin, cytoskeleton and cell cycle regulators [13] , [14] . The expression of PELP1 is deregulated in hormone-regulated cancers such as breast, ovarian and prostate [15] , [16] , with a two- to three-fold increase in protein expression observed in high-grade prostate tumours compared with normal or low-grade tumours [17] , [18] , [19] . Recently, our laboratory demonstrated that PELP1 has a critical role in AR-mediated genomic signalling in prostate cancer cells both in the absence and presence of androgenic ligand [20] . Examination of the PELP1 protein sequence reveals ten copies of a conserved LXXLL motif, also known as a nuclear receptor box, where L is leucine and X is any amino acid including leucine [14] . This short consensus LXXLL sequence is well established to be critical for interaction between nuclear receptors and coregulators that function to regulate receptor activity via a C-terminal ligand-binding domain (LBD) interaction [14] . AR specifically interacts with proteins presenting LXXLL motifs via its AF2 domain at the C terminus through a dimorphic cleft that enables interaction with amino-acid residues such as leucines in an α-helical conformation. Interactions between AR and proteins containing LXXLL motifs have been shown to be necessary and, in certain contexts, sufficient for AR-mediated transcriptional regulation [21] . Prior studies have shown that peptides derived from LXXLL motifs can block interactions between AR and cofactors containing LXXLL motifs [21] . The clinical utility and translatability of peptides reported to date have been limited by rapid metabolic degradation, low bioavailability, lack of oral activity and poor cell permeability. Consequently, critical PPIs such as the AR–AF2 interaction with coregulators have been deemed undruggable [22] . Peptidomimetics, also known as peptide mimetics, are small organic molecules that do not possess a peptide backbone structure, but retain a capacity to interact with the same target protein by arranging essential functional groups (that is, pharmacophores) into the required three-dimensional pattern complimentary to the binding pocket in the protein [23] . Peptidomimetics uniquely combine the advantages of both peptides (for example, high efficacy, target selectivity) and small organic molecules (for example, cell permeability, stability from protease-mediated proteolytic degradation, oral activity and bioavailability). In this study, we explored the rational design of LXXLL peptidomimetics and their effect on the interaction between AR and PELP1, AR signalling and the growth or survival of prostate cancer cells. We demonstrate the utility of the rational design strategy and believe that these data validate the importance of the interaction between AR and PELP1 in prostate cancer. Design and synthesis of the peptidomimetics D1 and D2 Evaluation of the crystallographic structure of a peptide containing the LXXLL sequence bound to AR shows that the LXXLL motif adopts an α-helical structure and that the side chains of the three leucines at the i , i +3 and i +4 positions interact with the hydrophobic pocket in the AF2 domain of AR [24] , [25] . We used the rigid and pre-organized structure of a bis-benzamide scaffold [26] to design the peptidomimetic D2 that mimics the LXXLL motif and disrupts the interaction between AR and NR box containing proteins such as PELP1 ( Fig. 1a ). Two isobutyl groups were used to reproduce the side chains at the i and i +4 positions of the LXXLL motif, creating a hydrophobic surface for interaction with AR ( Fig. 1b ). To validate its mimicry, the structure of D2 was studied by molecular mechanics using MacroModel (version 9.0, Schrödinger) [27] . A Monte Carlo conformational search was carried out using MM3 force field and a GB/SA solvation model [28] . The computational analysis demonstrated that the two isobutyl groups of the lowest energy conformation of D2 ( Fig. 1c ) overlaid well the side chains of the two leucines at the i and i +4 positions in the helical LXXLL motif ( Fig. 1c ). Molecular modelling and docking studies of AR and D2 using AutoDock (version 4.0, The Scripps Research Institute, La Jolla, CA) [29] illustrated an excellent fit between the D2 mimetic and the AF2 domain in the carboxy terminus of the AR; the two isobutyl groups of D2 recapitulate the hydrophobic interaction evident in the crystal structure of an AR-bound LXXLL peptide ( Fig. 1e ). 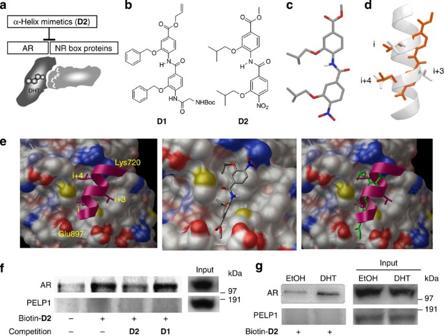Figure 1: Structural design and synthesis of the LXXLL peptidomimeticD2. (a)D2was structurally designed to disrupt the interaction between AR and NR box proteins containing the LXXLL motif such as PELP1. (b) Chemical structure of the bis-benzamide-based peptidomimeticD2(right) and its inactive relativeD1(left), and (c) the lowest energy conformation ofD2. (d) Overlay of the energy-minimizedD2(orange) over the α-helical LXXLL motif (white) (e) Docking studies ofD2on the AF2 domain of AR using AutoDock: Two isobutyl groups ofD2corresponding to the leucines at theiandi+4 positions of the LXXLL motif fit into the hydrophobic pocket in the AF2 domain in a manner similar to the known interactions between the LXXLL motifs and the AR. Crystal structure (PDB code 1T63) of the LXXLL motif bound on the AF2 domain (left).D2docked in the same binding pocket (middle). Superimposition of the dockedD2(green) over the crystal structure of the LXXLL motif (purple) (right). (f)D2directly binds to AR. The total cell lysate from C4-2 cells (200 μg), cultured in T-media with 10% FBS, was incubated with 1.5 nmoles of biotinylatedD2(Biotin-D2) alone or in the presence of tenfold excess unbiotinylatedD2(15 nmoles) or unbiotinylatedD1(15 nmoles). Input is shown in the right hand panel. (g) Effect of DHT onD2binding to AR: LNCaP cells were serum starved overnight in pfRPMI+3% CFS in the presence or absence of 10 nM DHT and the cell lysate collected. Immunoprecipitation experiments were performed usingBiotin-D2. Input lanes are also shown. Figure 1: Structural design and synthesis of the LXXLL peptidomimetic D2 . ( a ) D2 was structurally designed to disrupt the interaction between AR and NR box proteins containing the LXXLL motif such as PELP1. ( b ) Chemical structure of the bis-benzamide-based peptidomimetic D2 (right) and its inactive relative D1 (left), and ( c ) the lowest energy conformation of D2 . ( d ) Overlay of the energy-minimized D2 (orange) over the α-helical LXXLL motif (white) ( e ) Docking studies of D2 on the AF2 domain of AR using AutoDock: Two isobutyl groups of D2 corresponding to the leucines at the i and i +4 positions of the LXXLL motif fit into the hydrophobic pocket in the AF2 domain in a manner similar to the known interactions between the LXXLL motifs and the AR. Crystal structure (PDB code 1T63) of the LXXLL motif bound on the AF2 domain (left). D2 docked in the same binding pocket (middle). Superimposition of the docked D2 (green) over the crystal structure of the LXXLL motif (purple) (right). ( f ) D2 directly binds to AR. The total cell lysate from C4-2 cells (200 μg), cultured in T-media with 10% FBS, was incubated with 1.5 nmoles of biotinylated D2 ( Biotin-D2 ) alone or in the presence of tenfold excess unbiotinylated D2 (15 nmoles) or unbiotinylated D1 (15 nmoles). Input is shown in the right hand panel. ( g ) Effect of DHT on D2 binding to AR: LNCaP cells were serum starved overnight in pfRPMI+3% CFS in the presence or absence of 10 nM DHT and the cell lysate collected. Immunoprecipitation experiments were performed using Biotin-D2 . Input lanes are also shown. Full size image The synthesis of the peptidomimetic D2 and its analogues is detailed in the Supplementary Methods . Briefly, the peptidomimetic D2 was constructed by making an amide bond between methyl 4-amino-3-isobutoxybenzoate ( 2 ) and 3-isobutoxy-4-nitrobenzoyl chloride ( 4 ), both of which were prepared from a 3-isobutoxy-4-nitrobenzoic acid ( 1 ). Conversely, a bis-benzamide containing two benzyl groups ( D1 ) was synthesized as a control by following the previously reported procedure [30] . Initial evaluation indicated that the LXXLL peptidomimetic D2 was stable in DMSO at room temperature and −70 °C over 6 months of storage. Furthermore, the peptidomimetics were not toxic in cell culture within a concentration range of 10–200 nM as evidenced by cell viability assays ( Supplementary Fig. S1 ) in a variety of prostate ( n =6) cell lines. Incubation of cells with D2 revealed rapid uptake within minutes, as demonstrated by fluorescein-conjugated D2 (CF2-D2, Supplementary Fig. S2 ). Biotinylated D2 ( Biotin-D2 ) was able to pull down AR but not PELP1 following incubation with protein lysate from C4-2 cells and subsequently eluted from a streptavidin column ( Fig. 1f ). Binding of AR to Biotin-D2 is enhanced by the addition of 10 nM DHT ( Fig. 1g ). Further, unbiotinylated D2 but not unbiotinylated D1 could compete for the interaction between Biotin-D2 and AR ( Fig. 1f ). These data confirm the direct and specific binding of D2 to AR and that DHT enhances the binding of D2 to AR. D2 blocks the AR interaction with PELP1 Confirmation that D2 blocks PPIs between AR and LXXLL motif-containing coregulators was obtained from co-immunoprecipitation (co-IP) studies of AR and PELP1 ( Fig. 2a ). As shown previously, treatment of prostate cancer cells lines LAPC4, C4-2, VCaP and CWR22Rv1 with DHT enhanced the interaction between AR and PELP1 ( Fig. 2a , shown for LNCaP) [20] . Preincubation of LNCaP cells with increasing concentrations of D2 , but not D1 , blocked the interaction between AR and PELP1 even in the presence of DHT ( Fig. 2a ). D2 blocked AR–PELP1 interaction in a dose-dependent manner, with an IC 50 value of ~40 nM and complete inhibition of the complex formation at a dose of 200 nM. D2 was able to block interaction of AR with a subset of proteins containing LXXLL motifs, such as the heat shock protein (hsp27) ( Fig. 2a ). In contrast, D2 was not able to disrupt PPIs between AR and cofactors that lack the LXXLL motif such as importin beta, FoxA1, clusterin and hsp70 ( Supplementary Fig. S3 ). Also, the inability of D2 to block the interaction between PELP1 and oestrogen receptor-beta (ERβ) at these concentrations supports its specificity for AR interactions ( Fig. 2a ). The ability of D2 to block the AR–PELP1 interaction could be overcome by transient overexpression of either AR or PELP1 in a dose-dependent manner ( Fig. 2b ). These data strongly suggest that D2 blocks the interaction between AR and PELP1 by serving as a competitive antagonist to the interaction via the LXXLL motif. 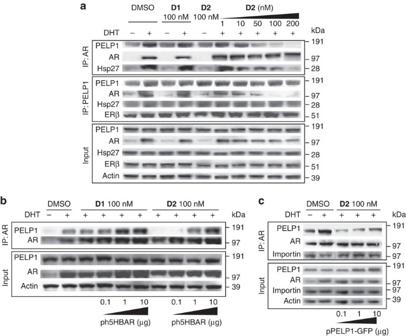Figure 2: D2 blocks AR protein–protein interactions with PELP1. (a) LNCaP cells were pretreated with DMSO,D1(100 nM) control or increasing concentrations ofD2(1, 10, 50, 100 and 200 nM) for 2 h and subsequently cultured in the presence or absence of 10 nM DHT for 24 h. Immunoprecipitation (IP) was performed by incubating cell lysates with specific antibodies for AR (top panel) or PELP1 (middle panel) and rabbit IgG DynaBeads for 60 min each at 4 °C. Immunocomplexes were resolved by SDS–polyacrylamide gel electrophoresis and blots hybridized with AR, PELP1, hsp27 and ERβ antibodies. Input is shown in the lower panel. Transient overexpression of (b) AR or (c) PELP1 by transfecting LNCaP cells with indicated amounts (in μg per well in a six-well plate) of corresponding expression plasmid rescuedD2(100 nM) -induced suppression of AR–PELP1 complex formation. Figure 2: D2 blocks AR protein–protein interactions with PELP1. ( a ) LNCaP cells were pretreated with DMSO, D1 (100 nM) control or increasing concentrations of D2 (1, 10, 50, 100 and 200 nM) for 2 h and subsequently cultured in the presence or absence of 10 nM DHT for 24 h. Immunoprecipitation (IP) was performed by incubating cell lysates with specific antibodies for AR (top panel) or PELP1 (middle panel) and rabbit IgG DynaBeads for 60 min each at 4 °C. Immunocomplexes were resolved by SDS–polyacrylamide gel electrophoresis and blots hybridized with AR, PELP1, hsp27 and ERβ antibodies. Input is shown in the lower panel. Transient overexpression of ( b ) AR or ( c ) PELP1 by transfecting LNCaP cells with indicated amounts (in μg per well in a six-well plate) of corresponding expression plasmid rescued D2 (100 nM) -induced suppression of AR–PELP1 complex formation. Full size image D2 blocks AR-dependent transcriptional activity Effect of D1 and D2 on AR-dependent transactivation was assessed by luciferase activity in LNCaP and LAPC4 cells transfected with ARE-luciferase reporter construct containing three copies of ARE upstream of a luciferase reporter ( Fig. 3a–c ). D1 had no influence on the AR transactivation, whereas D2 decreased DHT-induced activity back to basal levels in a dose-dependent manner ( Fig. 3c , shown for LNCaP cells). Again, overexpression of either AR ( Fig. 3a ) or PELP1 ( Fig. 3b ) was able to rescue the D2 -mediated suppression of DHT-induced transactivation ( Fig. 3a , shown for LAPC4 cells). 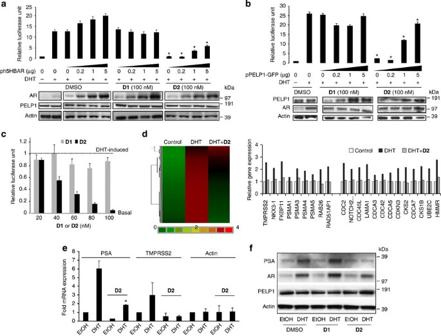Figure 3: D2 blocks AR transcriptional activity. LAPC4 cells were cotransfected with 0.5 μg of a minimal ARE-luciferase reporter construct containing three copies of ARE upstream of -luciferase reporter gene and indicated amounts (μg per well in a six-well plate) of plasmids encoding (a) AR (ph5HBAR) or (b) PELP1 (pPELP1-GFP). Cells were then pretreated with DMSO,D1(100 nM) orD2(100 nM) for 2 h followed by culture in the presence or absence of 10 nM DHT. Luciferase activity measured after 48 h shows that overexpression of AR or PELP1 can rescueD2suppression of DHT-induced AR transcriptional activity. Data are normalized to untreated cells and presented as relative luciferase units. Error bars represent the mean±s.d. *t-test,P<0.05 peptidomimetic treatment versus DHT alone. AR (~110 kDa) and PELP1 (~170 kDa) protein expression was visualized by immunoblot analysis of an independent set of cells treated in the same way. (c) Dose response ofD1andD2on ARE-luciferase activity: LNCaP cells were transfected with 0.5 μg of ARE-luciferase reporter construct and were treated with indicated concentrations (nM) ofD1orD2before treatment with 10 nM DHT. Luciferase activity was measured after 48 h and normalized to total protein concentration. (d) Left: gene expression profiling was performed in C4-2 cells treated with vehicle, DHT (10 nM) or DHT (10 nM)+D2(100 nM). Heat map display indicates thatD2blocked a majority of DHT-induced transcription. Right: expression levels of specific androgen-regulated genes and genes involved in cell proliferation in C4-2 cells treated with DHT (10 nM) orD2(100 nM)+DHT (10 nM) relative to untreated cells, as determined by gene expression profiling. The colour scale calibrates the fold differences in gene expression from baseline. (e) Validation of PSA and TMPRSS2 gene expression by QPCR analysis in an independent set of RNA. Actin mRNA level was used to demonstrate specificity of AR-regulated genes. Data is expressed as fold expression over untreated cells. Error bars represent the mean±s.d. of biological triplicates. *t-test,P<0.05D2versus DMSO. (f) Western blotting for PSA, AR and PELP1 in LAPC4 cells pretreated with DMSO,D1(100 nM) orD2(100 nM) for 2 h before the addition of 10 nM DHT. Actin was used as a loading control. Figure 3: D2 blocks AR transcriptional activity. LAPC4 cells were cotransfected with 0.5 μg of a minimal ARE-luciferase reporter construct containing three copies of ARE upstream of -luciferase reporter gene and indicated amounts (μg per well in a six-well plate) of plasmids encoding ( a ) AR (ph5HBAR) or ( b ) PELP1 (pPELP1-GFP). Cells were then pretreated with DMSO, D1 (100 nM) or D2 (100 nM) for 2 h followed by culture in the presence or absence of 10 nM DHT. Luciferase activity measured after 48 h shows that overexpression of AR or PELP1 can rescue D2 suppression of DHT-induced AR transcriptional activity. Data are normalized to untreated cells and presented as relative luciferase units. Error bars represent the mean±s.d. * t -test, P <0.05 peptidomimetic treatment versus DHT alone. AR (~110 kDa) and PELP1 (~170 kDa) protein expression was visualized by immunoblot analysis of an independent set of cells treated in the same way. ( c ) Dose response of D1 and D2 on ARE-luciferase activity: LNCaP cells were transfected with 0.5 μg of ARE-luciferase reporter construct and were treated with indicated concentrations (nM) of D1 or D2 before treatment with 10 nM DHT. Luciferase activity was measured after 48 h and normalized to total protein concentration. ( d ) Left: gene expression profiling was performed in C4-2 cells treated with vehicle, DHT (10 nM) or DHT (10 nM)+ D2 (100 nM). Heat map display indicates that D2 blocked a majority of DHT-induced transcription. Right: expression levels of specific androgen-regulated genes and genes involved in cell proliferation in C4-2 cells treated with DHT (10 nM) or D2 (100 nM)+DHT (10 nM) relative to untreated cells, as determined by gene expression profiling. The colour scale calibrates the fold differences in gene expression from baseline. ( e ) Validation of PSA and TMPRSS2 gene expression by QPCR analysis in an independent set of RNA. Actin mRNA level was used to demonstrate specificity of AR-regulated genes. Data is expressed as fold expression over untreated cells. Error bars represent the mean±s.d. of biological triplicates. * t -test, P <0.05 D2 versus DMSO. ( f ) Western blotting for PSA, AR and PELP1 in LAPC4 cells pretreated with DMSO, D1 (100 nM) or D2 (100 nM) for 2 h before the addition of 10 nM DHT. Actin was used as a loading control. Full size image We next examined whether D2 could block DHT-induced genomic activation of AR signalling using genome-wide microarray profiling ( Fig. 3d ). To do this, mRNA levels of genes in C4-2 and CWR22Rv1 cells treated with D2 for 2 h before DHT treatment were assessed relative to cells treated with DHT alone using the Illumina microarray system. Remarkably, D2 blocked a significant proportion of DHT-induced transcription, with inhibition of more than 1,500 of the 1,900 known DHT-regulated transcripts (79%) in C4-2 and CWR22Rv1 cells, including 219 of the 341 transcripts (64%) whose expression was increased more than twofold ( Fig. 3d , shown for C4-2 cells). Close examination of the microarray results revealed that D2 decreased the DHT-induced expression of classic AR-regulated genes TMPRSS2, NKX3.1, PSMA and kallikrein kinases, as well as critical proliferative genes such as cyclins and cyclin-dependent kinases ( Fig. 3d , right panel). These findings were validated independently at the RNA level using qRT–PCR evaluation of PSA and TMPRSS2 expression ( Fig. 3e ). While PSA and TMPRSS2 mRNA levels were decreased by D2 in the presence of DHT, mRNA levels of actin, a gene not regulated by AR, was unaffected by D2 ( Fig. 3e ). Although D2 was effective at blocking AR genomic activity, no effects were observed on DHT-induced non-genomic pathways such as Erk and Src phosphorylation ( Supplementary Fig. S4 ). Finally, D2 reduced the DHT-induced expression of the AR and PSA proteins in LNCaP and LAPC4 cells, while PELP1 protein levels were not altered by D1 or D2 ( Fig. 3f , shown for LNCaP). This decrease in AR and PSA protein levels was found to be consistent with the measured decrease in mRNA levels of AR ( Supplementary Fig. S5 ) and PSA further confirming that D2 inhibits the gene expression of these AR-regulated proteins. To evaluate the specificity of D2 for the C-terminal LBD of the AR, truncated versions of AR were used including the constitutively active ARv7 splice variant, which contains the AR N-terminal domain (NTD) and DNA-binding domain (DBD), but lacks the LBD, and a synthetic construct ARΔ1 that contains both the AR-DBD and LBD, but lacks the NTD ( Fig. 4a ). D2 inhibited both full-length AR activity and ARΔ1 activity, but was unable to inhibit ARv7 activity or CMV-βgal reporter activity ( Fig. 4b ). Immunoprecipitation studies indicate that PELP1 interacts with both full-length AR and ARΔ1 but not ARv7 and that D2 blocks this interaction ( Fig. 4c ). These data are consistent with the model that AR LBD is required for AR–PELP1 interaction, and that D2 blocks this interaction through the LBD. 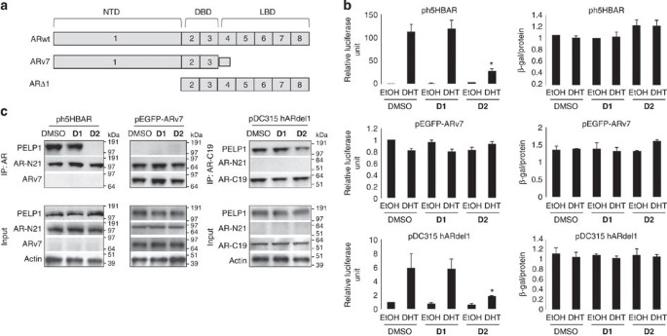Figure 4: D2 selectively inhibits AR LBD activity. (a) Schematic of full-length AR (ARwt), ARv7 and ARΔ1. Exons that code for the different domains (NTD, DBD and LBD) are indicated by numbers (1–8). (b) AR transcriptional activity (left) and CMVβgal activity (right) in PC3 cells transfected with 0.5 μg of expression plasmids for AR (ph5HBAR), ARv7 (pEGFP-ARv7) or ARΔ1 (pDC315 hARdel1) along with 0.3 μg each of ARE-luciferase reporter plasmid and pCMVβgal in P-60 dishes. Cells were trypsinized 24 h after transfection and plated on six-well dishes under serum-starvation conditions for 24 h. Cells were then treated with DMSO, 100 nMD1orD2for 2 h before treatment with 10 nM DHT for 48 h and luciferase and β-gal activity measured and normalized to total protein concentration. Fold changes were calculated relative activity in untreated cells. Data is representative of three independent experiments and is shown as mean±s.d., *P<0.05. (c) Cell lysate from DHT-treated transfected PC3 cells were subjected to immunoprecipitation using AR antibodies targeted against an epitope either in the N-terminal region of AR (AR-N21) or in the C-terminal region of AR (AR-C19), or a third antibody that is specific for ARv7 (ARv7). Molecular weight markers indicate AR full-length in lysates of PC3 cells transfected with p5HBAR (detected with AR-N21 antibody) and AR ~70 kDa in lysates of PC3 cells transfected with pEGFP-ARv7(detected with AR-N21 and ARv7 antibodies). The AR-C19 antibody detected an ~50-kDa protein in pDC315 hARdel1-transfected PC3 cells. Figure 4: D2 selectively inhibits AR LBD activity. ( a ) Schematic of full-length AR (ARwt), ARv7 and ARΔ1. Exons that code for the different domains (NTD, DBD and LBD) are indicated by numbers (1–8). ( b ) AR transcriptional activity (left) and CMVβgal activity (right) in PC3 cells transfected with 0.5 μg of expression plasmids for AR (ph5HBAR), ARv7 (pEGFP-ARv7) or ARΔ1 (pDC315 hARdel1) along with 0.3 μg each of ARE-luciferase reporter plasmid and pCMVβgal in P-60 dishes. Cells were trypsinized 24 h after transfection and plated on six-well dishes under serum-starvation conditions for 24 h. Cells were then treated with DMSO, 100 nM D1 or D2 for 2 h before treatment with 10 nM DHT for 48 h and luciferase and β-gal activity measured and normalized to total protein concentration. Fold changes were calculated relative activity in untreated cells. Data is representative of three independent experiments and is shown as mean±s.d., * P <0.05. ( c ) Cell lysate from DHT-treated transfected PC3 cells were subjected to immunoprecipitation using AR antibodies targeted against an epitope either in the N-terminal region of AR (AR-N21) or in the C-terminal region of AR (AR-C19), or a third antibody that is specific for ARv7 (ARv7). Molecular weight markers indicate AR full-length in lysates of PC3 cells transfected with p5HBAR (detected with AR-N21 antibody) and AR ~70 kDa in lysates of PC3 cells transfected with pEGFP-ARv7(detected with AR-N21 and ARv7 antibodies). The AR-C19 antibody detected an ~50-kDa protein in pDC315 hARdel1-transfected PC3 cells. Full size image D2 prevents AR nuclear translocation We then evaluated if D2 could affect DHT-induced translocation of AR from the cytoplasm to the nucleus using two distinct approaches. Evaluation of real-time nuclear localization of exogenously transfected GFP-tagged AR after 1 nM DHT treatment in the presence of 100 nM D1 or D2 using fluorescence microscopy revealed that pretreatment with D2 blocked DHT-induced translocation of AR to the nucleus compared with the control D1 or DMSO ( Fig. 5a ). Additionally, endogenous AR levels in biochemically enriched cytoplasmic and nuclear fractions were consistent with D2 reducing DHT-induced translocation and stabilization of AR in the nucleus compared with treatment with the control D1 or DMSO ( Fig. 5b ). 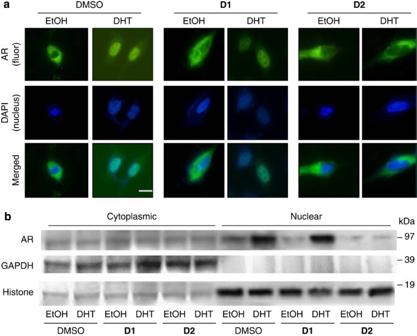Figure 5: D2 prevents AR nuclear translocation. (a) Fluorescence microscopy on LNCaP cells transiently transfected with AR-GFP that were pretreated with DMSO, 100 nMD1orD2before treatment with 1 nM DHT for 4 h. Green stain is AR (GFP) and blue stain is DAPI (for nucleus). Scale bar, 2.5 microns. (b) Nuclear and cytoplasmic extracts were collected from LNCaP cells pretreated with 100 nMD1orD2for 2 h followed by 10 nM DHT treatment for 16 h and subjected to western blot analysis. GAPDH was used as control for the cytoplasmic fraction and Histone H3 was used as control for the nuclear fraction. Figure 5: D2 prevents AR nuclear translocation. ( a ) Fluorescence microscopy on LNCaP cells transiently transfected with AR-GFP that were pretreated with DMSO, 100 nM D1 or D2 before treatment with 1 nM DHT for 4 h. Green stain is AR (GFP) and blue stain is DAPI (for nucleus). Scale bar, 2.5 microns. ( b ) Nuclear and cytoplasmic extracts were collected from LNCaP cells pretreated with 100 nM D1 or D2 for 2 h followed by 10 nM DHT treatment for 16 h and subjected to western blot analysis. GAPDH was used as control for the cytoplasmic fraction and Histone H3 was used as control for the nuclear fraction. Full size image D2 inhibits AR-mediated prostate cancer cell proliferation As D2 is a potent inhibitor of AR signalling ( Figs 3 and 5 ), we examined the effect of the LXXLL peptidomimetic on proliferation of prostate cancer cells using an MTT assay. Pretreatment with D2 prevented DHT-induced proliferation of a variety of AR-positive prostate cancer cell lines, including LNCaP, LAPC4, C4-2, RWPE-1, CWR22Rv1 and VCaP, but not AR-negative prostate cancer cell line PC3 ( Fig. 6a ). These data were confirmed using a CyQuant cell proliferation assay ( Fig. 6b , shown for LNCaP). The inhibition of cell proliferation by D2 was DHT-specific, as D2 had no effect on EGF-induced prostate cancer cell proliferation ( Supplementary Fig. S6 ). The inhibition of cell proliferation by D2 was dose-dependent with an IC 50 value of ~40 nM ( Fig. 6c ). The importance of the interaction between PELP1 and AR for DHT-mediated proliferation of prostate cancer cells was confirmed using rescue experiments, where D2 suppression of DHT-mediated cell proliferation was overcome by overexpression of PELP1 in LNCaP cells ( Fig. 6d ). That the effect of D2 on proliferation was mediated by an intracellular action of D2 was further corroborated by the findings that only the fluorescein-conjugated version of D2 (CF2- D2 ) that could enter the cell blocked DHT-induced proliferation of LNCaP cells ( Supplementary Fig. S2 ). 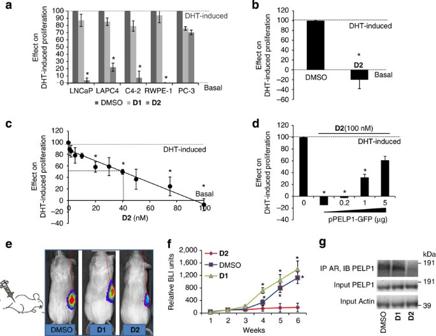Figure 6: D2 inhibits prostate cancer cell growthin vitroandin vivo. (a) A panel of prostate cancer cells pretreated with DMSO, 100 nMD1orD2for 2 h before 10 nM DHT treatment for 72 h were assessed by MTT proliferation assay. Data were normalized to the DMSO treatment for each cell line. (b) Effect of pretreatment with 100 nM ofD1andD2on DHT-induced proliferation in LNCaP cells by CyQuant assay. (c) Dose–response curve ofD2on the proliferation of LAPC4 cells. (d) Rescue of DHT-induced proliferation by overexpression of PELP1 by transfecting LNCaP cells with increasing amounts of pPELP1-GFP following suppression with 100 nMD2. (e) Subcutaneous C4-2 tumours were allowed to establish in SCID mice until palpable and detected on BLI. The basal rate of growth of these tumours was established for 1 week, followed daily intratumoural (i.t.) injections of DMSO, 10 mMD1orD2dissolved in 100 μl of 5% dextrose for 5 weeks. Effects on tumor growth were serially followed by BLI (shown ineafter 5 weeks of daily i.t. injections) and graphically represented as fold change±s.d. over bioluminescence measured at the start of treatment (f). (g) AR was immunoprecipitated from mouse tumors by incubating extracts with an AR antibody conjugated to rabbit IgG DynaBeads for 60 min at 4 °C. Immunocomplexes were resolved by SDS–polyacrylamide gel electrophoresis and blots hybridized for AR, PELP1 and actin. Input is shown in the lower panels. Data ina–dandfare representative of three independent experiments and is shown as mean±s.d., *P<0.05. Figure 6: D2 inhibits prostate cancer cell growth in vitro and in vivo . ( a ) A panel of prostate cancer cells pretreated with DMSO, 100 nM D1 or D2 for 2 h before 10 nM DHT treatment for 72 h were assessed by MTT proliferation assay. Data were normalized to the DMSO treatment for each cell line. ( b ) Effect of pretreatment with 100 nM of D1 and D2 on DHT-induced proliferation in LNCaP cells by CyQuant assay. ( c ) Dose–response curve of D2 on the proliferation of LAPC4 cells. ( d ) Rescue of DHT-induced proliferation by overexpression of PELP1 by transfecting LNCaP cells with increasing amounts of pPELP1-GFP following suppression with 100 nM D2 . ( e ) Subcutaneous C4-2 tumours were allowed to establish in SCID mice until palpable and detected on BLI. The basal rate of growth of these tumours was established for 1 week, followed daily intratumoural (i.t.) injections of DMSO, 10 mM D1 or D2 dissolved in 100 μl of 5% dextrose for 5 weeks. Effects on tumor growth were serially followed by BLI (shown in e after 5 weeks of daily i.t. injections) and graphically represented as fold change±s.d. over bioluminescence measured at the start of treatment ( f ). ( g ) AR was immunoprecipitated from mouse tumors by incubating extracts with an AR antibody conjugated to rabbit IgG DynaBeads for 60 min at 4 °C. Immunocomplexes were resolved by SDS–polyacrylamide gel electrophoresis and blots hybridized for AR, PELP1 and actin. Input is shown in the lower panels. Data in a – d and f are representative of three independent experiments and is shown as mean±s.d., * P <0.05. Full size image D2 inhibits AR-dependent growth of xenograft tumours in vivo The effect of the peptidomimetic D2 in vivo was evaluated using prostate cancer xenograft models. Initial toxicity experiments showed no systemic toxicity, induction of hepatic microsomes ( Supplementary Fig S7 ) or changes in the weight of the mice ( n =6) at 6 weeks following intraperitoneal administration of D2 at concentrations up to 100 mg kg −1 . Direct intratumoural injections of DMSO (vehicle control), D1 or D2 were administered to established subcutaneous xenografts of C4-2 cells and their growth followed serially by bioluminescence imaging (BLI). Whereas the tumours continued to grow despite injections with D1 or DMSO, administration of D2 significantly blocked tumour growth as evidenced by decreased BLI ( Fig. 6e ). D2 did not appear to be cytotoxic to the prostate cancer cells, but was cytostatic. Assessment of the tumours derived from these mice revealed that target inhibition was achieved, as AR–PELP1 complex formation was blocked in D2 -treated animals but could be readily detected in tumours injected with D1 or DMSO ( Fig. 6g ). Additionally, intraperitoneal injections of D2 but not D1 or DMSO blocked the growth of these subcutaneous C4-2 xenografts over 4 weeks ( Supplementary Fig. S8 ). D2 inhibits AR expression in human tumours cultured ex vivo In explant cultures ( n =7) derived from freshly extirpated high-risk, high-volume human primary prostate cancer specimens ( Fig. 7a ), culture with D2 , but not D1 or DMSO blocked the interaction between AR and PELP1 as evidenced in co-IP assays ( Fig. 7b ). Most importantly, D2 decreased AR nuclear immunostaining in the prostate cancer tissues when compared to D1 or DMSO controls ( Fig. 7c ). The reduction in total AR immunostaining in these ex vivo cultures was similar to that observed for the AR-antagonist MDV3100 ( Fig. 7d ). These data are consistent with the ability of D2 to block AR nuclear translocation and or modulate ligand-induced receptor stabilization and chromatin binding. 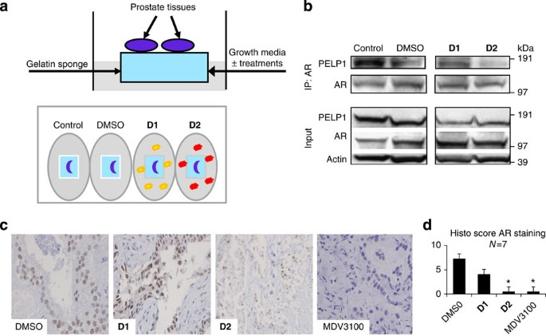Figure 7: D2 inhibits AR–PELP1 interaction in prostate cancer cell explants. (a) Following radical prostatectomy, the extirpated prostate is bivalved and a core of tissue corresponding to the area of the tumour is removed by the pathologist. The tissue is then transferred to the laboratory and dissected into 1 mm3fragments. The fragments are then cultured on gelatin sponge submerged in media supplemented with 10% fetal calf serum. Following incubation with media for a defined time period (2 days), the explants are then processed for further evaluation. (b) Immunoprecipitation (IP) analyses of these prostate explants demonstrate the PPIs between AR and PELP1 in the presence ofD1, DMSO but notD2(100 nM). (c) Representative AR immunohistochemistry (IHC) staining in prostate cancer explants following incubation for 2 days in either complete media in the presence of 100 nM DMSO,D1,D2or 10 μM of MDV3100 reveals thatD2blocks nuclear AR expression. (d) Quantitation of AR immunostaining in prostate explants is shown for DMSO,D1,D2or MDV3100 as a control (P<0.05). Data is shown as mean±s.d.,n=7, *P<0.05. Figure 7: D2 inhibits AR–PELP1 interaction in prostate cancer cell explants. ( a ) Following radical prostatectomy, the extirpated prostate is bivalved and a core of tissue corresponding to the area of the tumour is removed by the pathologist. The tissue is then transferred to the laboratory and dissected into 1 mm 3 fragments. The fragments are then cultured on gelatin sponge submerged in media supplemented with 10% fetal calf serum. Following incubation with media for a defined time period (2 days), the explants are then processed for further evaluation. ( b ) Immunoprecipitation (IP) analyses of these prostate explants demonstrate the PPIs between AR and PELP1 in the presence of D1 , DMSO but not D2 (100 nM). ( c ) Representative AR immunohistochemistry (IHC) staining in prostate cancer explants following incubation for 2 days in either complete media in the presence of 100 nM DMSO, D1 , D2 or 10 μM of MDV3100 reveals that D2 blocks nuclear AR expression. ( d ) Quantitation of AR immunostaining in prostate explants is shown for DMSO, D1 , D2 or MDV3100 as a control ( P <0.05). Data is shown as mean±s.d., n =7, * P <0.05. Full size image AR requires interactions with its coregulator proteins to actively engage in transcriptional activity [31] , [32] . Given that many coregulators interact with the AR through motifs containing the consensus LXXLL motif [24] , where L is Leucine and X is any amino acid, we rationally designed peptidomimetics that imitate the LXXLL motif with the aim of disrupting necessary AR-mediated PPIs and thereby inhibit AR signalling and the survival of prostate cancer cells. Previous attempts to generate LXXLL-based peptide drugs have been unsuccessful, predominantly due to issues with cell permeability and degradation. Recently, we have developed oligo-benzamide scaffolds that can place two or three substituents corresponding to the side chains of amino-acid residues found at the i , i +4 and i +7 positions of an α-helix, as they appear in the helix, effectively mimicking one helical face [26] . Since our initial report in 2007 (ref. 26 ), the ability of the oligo-benzamide scaffolds to mimic helical structures and disrupt PPIs have been further established [33] , [34] , [35] , [36] . We also demonstrated that the oligo-benzamide-based peptidomimetics can easily be synthesized by using simple and uncomplicated reactions with high yields [30] . In this study, we examined the effect of D2 primarily on the interaction between AR and PELP1 as the paradigm for interactions between AR and LXXLL-containing coregulators. Our data show that the peptidomimetic D2 effectively disrupts the interaction between AR and LXXLL-containing cofactors with an IC 50 in the nM range. Interestingly, the interaction between AR and several other known LXXLL-containing proteins, including SRC-1, hsp90, hsp70, was not affected by D2 . This suggests that those proteins may interact with AR via alternative domains or possess a higher binding affinity to AR relative to D2 . It also is possible that D2 restricts AR interaction with a specific conformation of the LXXLL domains that is found only in a subset of coregulators. Further studies are needed to determine the complete repertoire of interactions that are blocked by the LXXLL peptidomimetic D2 . One major advantage of D2 is its ability to block DHT-induced nuclear translocation and or stability of AR. To date, the only clinically available agent that has the capability to block DHT-induced nuclear translocation is the AR-antagonist MDV3100 (ref. 37 ), which has recently been approved by the FDA for use in post-chemotherapy CRPC patients [38] , [39] , [40] . Collectively, our data suggests that D2 prevents AR nuclear translocation by blocking its interaction with proteins involved in nuclear transport, congruent with our previously postulated role of PELP1 [20] . These data also indicate that D2 and its analogues may assist with delineating the relative contribution of putative factors involved in AR nuclear translocation. Additionally, we note that other modes of action of D2 cannot be excluded, such as disruption of AR genomic function by reducing either AR stability or residency time on chromatin, and/or enhancing nuclear export and subsequent receptor degradation. D2 blocks the DHT-induced genomic activity of AR in prostate cancer cells with high efficacy (IC 50 value of 40 nM). This effect of D2 could be rescued by overexpression of either AR or PELP1, suggesting that D2 works as a competitive inhibitor of AR function. Consistent with this finding, the inhibitory activity of D2 resulted in growth suppression in AR-positive but not AR-negative prostate cancer cells. Additionally, our studies in vivo demonstrated cytostatic effects of D2 in xenograft prostate tumours, and we provide evidence using human tumour ex vivo culture that D2 can access prostate tumour cells in their native environment to achieve target modulation. Taken together, these data strongly suggest that D2 is clinically translatable. Critically, the documented ability of D2 to block DHT-induced genomic activation makes it an attractive candidate for further development as a therapeutic agent. The primary limitation of a peptidomimetic strategy that mimics the LXXLL motif is the potential for a large number of PPIs to be disrupted, including those involving other steroid receptors. The broad targeting of multiple pathways may enable effective targeting of cancer cells, as demonstrated by the success of agents targeting multiple kinase pathways, [41] , [42] but may also result in toxicity, which would limit its clinical utility. In our tests to date, no significant toxicity has been noted across a large range of cell lines or upon oral, intratumoural or intraperitoneal administration in animals over long time periods of administration. Further, the peptidomimetic D2 is based on the bis-benzamide platform that allows for presentation of only two binding sites from helical motifs. Consequently, D2 likely blocks a large subset of interactions involving the LXXLL motif. Refinements to the specificity of targeting may be achieved by using larger oligo-benzamide scaffolds that can accommodate an increased number of binding elements from the same helical secondary structure and thus block fewer PPIs through the LXXLL motif. Finally, these data support a critical role for PELP1 in AR-driven genomic signalling. The overlap between the IC 50 values for both D2 -mediated disruption of AR–PELP1 interaction and DHT-induced genomic function and proliferation strongly supports this hypothesis. The ability of overexpression of PELP1 to rescue the D2 -mediated knockdown of DHT-induced gene expression or proliferation bears testament to its central regulatory role in prostate cancer cells. Importantly, because PELP1 has ten copies of the consensus LXXLL motif, its interactions with AR may be more susceptible to this peptidomimetic-based approach. Based on our results, further studies to validate the utility of D2 as a therapeutic agent for prostate cancer are warranted. Materials The compound D1 was prepared as reported previously [30] . The compound D2 was synthesized from a 3-hydroxy-4-nitrobenzoic acid through a series of reactions including O -alkylation of 3-hydroxy-4-nitrobenzoate, reduction of the nitro group, hydrolysis of the ester, and amide bond formation ( Supplementary Methods ). The NMR and MS characterizations are also detailed ( Supplementary Fig. S9 ). Molecular docking of D2 AutoDock 4.2 software package was used to dock D2 to the AR ( Supplementary Methods ). Cell lines and culture LNCaP and PC3 cells were obtained from the American Type Culture Collection (ATCC, Manassas, VA). LNCaP, C4-2 and PC3 were maintained in T medium (Invitrogen, Carlsbad, CA) supplemented with 5% fetal bovine serum (FBS); CWR22Rv1, obtained from Dr ChingHai Kao (Indiana University), was maintained in Dulbecco’s Modified Eagle’s Medium (DMEM) (Mediatech, Manassas, VA) containing 10% FBS; LAPC4 cells, obtained from Dr Charles Sawyer (UCLA), were maintained in Iscove’s DMEM (Mediatech, Manassas, VA) containing 10% FBS. All growth media were supplemented with penicillin (100 IU ml −1 ) and streptomycin (100 μg ml −1 ). Plasmid constructs Plasmid constructs for full-length AR, ph5HBAR (AR cDNA cloned into pCMV5 expression vector), was provided by Dr Scott Dehm (University of Minnesota) and full-length PELP1, pPELP1-GFP (PELP1 cloned into pAcGFP1-C1 vector), by Dr Ratna Vadlamudi (University of Texas Health Science Center at San Antonio). Plasmid for ARE-luciferase, constructed by inserting three copies of androgen response region (−244 to −96 bp) of rat probasin gene upstream of tk-luc reporter in pT81luc, was a gift from Dr Robert J Matusik (Vanderbilt University Medical Center). Plasmid for CMV-βgal was provided by Dr Leland Chung (Cedars Sinai Medical Center, Los Angeles). pEGFP-ARv7, which contains the full-length AR-v7 cDNA inserted into pEGFP-C3, was a gift from Dr Jun Luo (John Hopkins University). pcDNA3.1-ARv567es was kindly provided by Dr Stephen Plymate (University of Washington, Seattle). Plasmid for ARΔ1 (pDC315 hARdel1) that encodes AR without exon 1 at the NTD was provided by Dr Pekka Kallio. Androgen deprivation The cells were washed with PBS and the growth medium changed to phenol-red-free RPMI 1640 with 1–5% charcoal-stripped fetal bovine serum (CSF) for 48 h before treatment. Antibodies and reagents The AR and β-actin antibodies were purchased from Sigma (St Louis, MO); PELP1 antibody from Bethyl Laboratories (Montgomery, TX); AR-C19, GAPDH, Histone H3, tERK, tSrc, tAkt, ERβ and PSA antibodies from Santa Cruz Biotechnology (Santa Cruz, CA). pAkt, pSrc (T262/Y204) and pSrc (Y416) from Cell Signaling Technology (Danvers, MA). DHT was purchased from Sigma-Aldrich (St Louis, MO) and dissolved in ethanol. The synthetic androgen R1881 was purchased from Perkin Elmer (Boston, MA) and dissolved in ethanol. MDV3100 was purchased from Selleckchem (Houston, TX) and dissolved in DMSO. Proliferation assays Cells were plated (2–10 × 10 3 per well) in 96-well plates and subjected to androgen deprivation for 48 h as described above. Cells were pretreated with DMSO (vehicle control), D1 or D2 for 2 h. Media containing ethanol (vehicle control) or DHT was then added to a final concentration of 10 nM and cells cultured for another 72 h. Cell proliferation was measured using the MTT colorimetric assay (Roche Diagnostics, Indianapolis, IN) or CyQuant Cell proliferation assay (Invitrogen). All experiments were performed in triplicate and the average of experiments displayed. Fluorescein-conjugated peptidomimetics LNCaP cells were plated in six-well plates (1 × 10 4 per well) in T-media +5% FBS and allowed to attach for 24 h. Cells were then treated with one of two fluorescein-conjugated D2 peptidomimetics (at 100 μM): CF1- D2 ( D2 with fluorescein conjugated at the N terminus) or CF2- D2 ( D2 with fluorescein conjugated at the C terminus) for 4 h and observed under fluorescence microscope. Proliferation assays with these fluorescein-conjugated peptidomimetics were performed as described above for D2 . Western blot and immunoprecipitation analyses After treatments as indicated, total cellular protein was extracted and western blotting and/or immunoprecipitation analyses using Protein G Dynabeads (Invitrogen) were performed as previously described [20] . Binding assay Whole-cell lysate of C4-2 cells cultured in T-media +5% FBS was extracted using protein lysis buffer as described above. The cell lysate (200 μg) was incubated with 1.5 nM of Biotin-D2 dissolved in DMSO for 8 h at 4 °C with gentle rotation to allow binding. Streptavidin Dynabeads (150 μl, Invitrogen) were blocked in 2% BSA in PBS for 15 min and then incubated with the Biotin-D2 -lysate mixture at 4 °C overnight with gentle rotation. For competition assay, the cell lysate was incubated with Biotin-D2 in the presence of tenfold excess unbiotinylated D2 (15 nM) or unbiotinylated D1 (15 nM). Bead-lysate mixture not incubated with Biotin-D2 was used as negative control. Bound proteins were eluted by boiling sample in SDS loading buffer (New England Bioloabs, Ipswich, MA) for 10 min and separated on a polyacrylamide gel for analysis by western blot. RNA isolation and real-time reverse transcription–PCR Total cellular RNA was extracted with the RNeasy mini kit according to the manufacturer’s instructions (Qiagen, Valencia, CA). Complementary DNA (cDNA) was then synthesized from 1 μg RNA using the cDNA synthesis kit (Bio-Rad, Hercules, CA). PCR was performed on 2.5 μl cDNA using iQ SYBR Green Supermix (Bio-Rad) on an iCycler thermal cycler (Bio-Rad) with a denaturation step at 95 °C for 3 min followed by 40 cycles of amplification at 95 °C for 30 s, 60 °C for 30 s, and 72 °C for 60 s. Primer sequences are detailed in Supplementary Table S1 . All samples were performed in duplicates and experiments repeated at least twice. Data were normalized to 18S rRNA and fold induction determined using the ΔCt method. Gene expression profiling Total cellular RNA was extracted as described above from C4-2 and CWR22Rv1 cells pretreated with DMSO/ D2 (100 nM) for 2 h before EtOH/DHT (10 nM) treatment. Hybridization to HumanHT-12 v4 Bead Chip (Illumina) was performed at the UT Southwestern Microarray Core Facility according to manufacturer’s specifications. Transcript mRNA levels were measured using HiScan SQ (Illumina). The effect of peptidomimetics on the expression of known AR-responsive genes was evaluated. Data is presented as mRNA level in peptidomimetic-treated cells relative to untreated cells. The statistical analysis was performed for each gene separately by fitting the following analysis of variance model. Estimates of fold change were calculated, and genes with P -value<0.05, fold change>2, and average spot intensity>100 were further evaluated. Data analysis was performed and heat maps were generated using the statistical software Cluster 3.0 ( http://bonsai.hgc.jp ). Extraction of nuclear and cytoplasmic fractions Fractionation and extraction of nuclear and cytoplasmic proteins from LNCaP cells pretreated with 100 nM D1 or D2 before 10 nM DHT treatment for 16 h was performed using NE-PER Nuclear and Cytoplasmic Extraction Reagents (ThermoScientific, IL) according to manufacturer’s protocol. Luciferase assay Cells were transfected as indicated with Lipofectamine Plus (Invitrogen), then equally divided into 24-well plates and allowed to attach. The culture medium was replaced after 24 h with androgen deprivation medium containing DHT or vehicle control for 48 h. All experiments were performed in triplicate. Luciferase activity was measured using the Dual Luciferase assay system (Promega, Madison, WI) and normalized to sample protein concentration. Results are presented as fold change over untreated cells. Xenograft experiments Six-week-old SCID mice were subcutaneously inoculated with 2.5 × 10 6 C4-2 cells and tumours were allowed to establish. Treatment was initiated when mean tumour volume reached ~250 mm 3 and detectable on BLI. Mice received either DMSO or 10 mM D1 or 10 mM D2 (6 mice per treatment group) dissolved in 100 μl of 5% dextrose intratumourally every day for 5 weeks, and the tumour growth followed by BLI. Results are presented as fold change over bioluminescence measured at the start of treatment. Human explant experiments Fresh prostate cancer tissues were obtained with informed consent from men undergoing radical prostatectomy at the Hospitals of the University of Texas Southwestern Medical Center (Dallas, TX) [43] (see Supplementary Table S2 for clinicopathological characteristics). The tissues were dissected into 1 mm 3 pieces and randomly placed in triplicates on a pre-soaked 1-cm 3 veterinary dental sponge (Novartis, East Hanover, NJ) inside the wells of a 12-well plate containing 600 μl RPMI 1640 with 5% heat-inactivated FBS, 100 units per ml penicillin-streptomycin and vehicle (DMSO) alone, D1 (100 nM) or D2 (100 nM). Tissues were cultured at 37 °C for 48 h and then formalin-fixed and paraffin embedded for immunohistochemistry analyses. Immunohistochemical staining We performed immunohistochemical staining for AR using serial sections from the paraffin-embedded blocks as described previously [20] . Optimum primary antibody dilutions were predetermined, using a prostate cancer as positive control sample for AR (polyclonal rabbit, N-20, dilution 1:50; Santa Cruz). Immunohistochemical analysis and scoring were done by a staff pathologist (PK) as previously described [20] . Statistical analysis All error bars represent mean±s.d. Student’s two-tailed t -test was used for the determination of statistical relevance between groups with P <0.05 considered as significant. How to cite this article: Ravindranathan, P. et al . Peptidomimetic targeting of critical androgen receptor–coregulator interactions in prostate cancer. Nat. Commun. 4:1923 doi: 10.1038/ncomms2912 (2013).